In situ copper faceting enables efficient CO2/CO electrolysis The copper (Cu)-catalyzed electrochemical CO 2 reduction provides a route for the synthesis of multicarbon (C 2+ ) products. However, the thermodynamically favorable Cu surface (i.e. Cu(111)) energetically favors single-carbon production, leading to low energy efficiency and low production rates for C 2+ products. Here we introduce in situ copper faceting from electrochemical reduction to enable preferential exposure of Cu(100) facets. During the precatalyst evolution, a phosphate ligand slows the reduction of Cu and assists the generation and co-adsorption of CO and hydroxide ions, steering the surface reconstruction to Cu (100). The resulting Cu catalyst enables current densities of > 500 mA cm −2 and Faradaic efficiencies of >83% towards C 2+ products from both CO 2 reduction and CO reduction. When run at 500 mA cm −2 for 150 hours, the catalyst maintains a 37% full-cell energy efficiency and a 95% single-pass carbon efficiency throughout. Renewable electricity powered CO 2 reduction (CO 2 R) to multicarbon (C 2+ ) products is a promising approach to carbon recycling, and an attractive alternative to fossil fuel reliant pathways. Copper is the only monometallic catalyst capable of catalyzing CO 2 to C 2+ products, and its crystal facets have been known to exert a significant influence on the CO 2 R activity and selectivity [1] , [2] , [3] , [4] . Specifically, the thermodynamically favorable Cu(111) facet favors C 1 production, whereas Cu(100) is active for C-C coupling [2] , [3] , [5] . To date, previous works in facet-controlled synthesis of Cu(100) catalysts mostly relied on colloidal synthesis using capping agents [6] , [7] , [8] that modulate the relative energy of facets during synthesis. However, organic additives often play impact the catalytic performance [9] and the resulting well-defined Cu catalysts such as Cu(100) nanocubes are prone to reconstruct during electrolysis [7] , [10] , [11] . One approach to bridge the demands of catalyst fabrication and performance testing is to use the same intermediate species throughout. This improves compatibility between synthesis and catalysis, and potentially sidesteps the challenges of catalyst reconstruction during electrolysis. To realize such an approach, the electrochemical reduction of Cu-based compounds offers one avenue to enable in situ growth of active sites [12] , [13] , [14] , [15] . CO 2 molecules are easily activated on the catalyst surface under negative potentials, in which the reduced intermediate species, such as CO, has strong interaction with Cu [16] , [17] and can play a role analogous to that of capping agents to direct the in situ growth of active Cu(100) during CO 2 R [13] . However, in situ reduction of traditional copper compounds is relatively fast and typically completed in less than five minutes [13] , [14] , [18] , [19] – an insufficient time for generating reduced intermediates at high coverages to direct crystal growth. As a result, the thermodynamically favorable Cu(111) facet is preferably exposed over Cu(100) (Fig. 1a ), and C 2+ production rates are low (<200 mA cm −2 ) from CO 2 R operated in a zero-gap membrane electrode assembly (MEA) electrolyzer [13] , [18] . Technoeconomic assessments suggest that production rates exceeding 300 mA cm −2 are essential for commercial viability [20] , [21] , [22] , and motivate a new approach to catalyst synthesis. Fig. 1: Schematic illustration and DFT prediction of the Cu faceting process. a Schematics of the in situ Cu(111) formation from weak CO adsorption during CO 2 R. b Schematics of the in situ Cu(100) formation from the co-adsorption of CO&OHˉ during CO 2 R. c The surface energies of Cu(111) and Cu(100) at different CO* and OHˉ surface coverages. d A contour plot of the surface energy difference between Cu(100) and Cu(111) by changing the surface coverages of CO* and OHˉ. e , Wulff construction clusters of copper without and with (co-)adsorption of CO* and OHˉ. Full size image We took the view that hydroxide ions on or near the copper surface can lower the CO 2 activation energy barrier and facilitate CO adsorption near the OH moiety [23] , [24] , [25] . Introducing OHˉ in a Cu precatalyst has also been shown to promote the growth of Cu(100) [26] , yet rapid OHˉ loss from the Cu surface via electroreduction results in a surface with Cu(100) and Cu(111) facets in similar proportion. We posited that the buildup of stable CO and OHˉ (CO&OHˉ) on Cu could promote the in situ synthesis of Cu(100)-rich catalysts compatible with efficient CO 2 electrolysis to multicarbon products (Fig. 1b ). Here we report an in situ copper faceting strategy to enable preferential exposure of Cu(100), accelerating electrosynthesis of C 2+ from both CO 2 R and COR. We introduce a phosphate ligand that facilitates CO&OHˉ co-adsorption on Cu during electrolysis. The subsequent interactions between CO&OHˉ and Cu guide the surface evolution, thereby favoring Cu(100) growth. We integrate the resulting Cu(100)-rich catalyst into a MEA electrolyzer and demonstrate a CO 2 -to-C 2+ conversion system with a Faradaic efficiency (FE) of 83% at 500 mA cm −2 . The catalyst also shows excellent performance from CO electrolysis, which enables single-pass carbon efficiency (SPCE) of 95%, full-cell energy efficiency (EE) of 41%, FE of 93%, and partial current density of 465 mA cm −2 towards C 2+ products. The Cu(100)-rich catalyst is also stable, providing sustained performance for an initial 150 operating hours. Density functional theory (DFT) calculations We began by assessing the surface coverage effect of CO* and OHˉ on the surface energies of Cu(111) and Cu(100) using DFT (Fig. 1c , Supplementary Figs. 1 – 6 ), in which there is no adsorbate-adsorbate interaction when calculating the surface energy. For the bare Cu, the calculated surface energies of Cu(111) and Cu(100) are 1.33 J m −2 and 1.47 J m −2 , respectively, suggesting that Cu(111) is the most stable facet in polycrystalline Cu, consistent with previous reports [13] , [27] . With the increase of CO* coverage, we found that the surface energies of Cu(111) and Cu(100) were both decreased, in which Cu(111) was favored over Cu(100) across a broad range of CO coverage from 0 ML to 4/9 ML. Thus despite an increase in the proportion of Cu(100) coverage, Cu(111) remains dominant in copper catalysts that are in situ synthesized using single CO 2 R intermediates (e.g. CO) – a finding consistent with the literature [13] , [18] , [19] . In contrast, the effect of OHˉ on Cu(100) formation is distinct; at an OHˉ coverage exceeding 2/9 ML, Cu(100) growth became more favorable over Cu(111) formation. 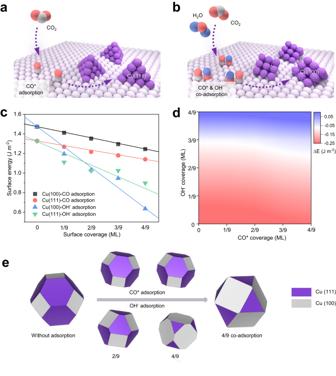Fig. 1: Schematic illustration and DFT prediction of the Cu faceting process. aSchematics of the in situ Cu(111) formation from weak CO adsorption during CO2R.bSchematics of the in situ Cu(100) formation from the co-adsorption of CO&OHˉ during CO2R.cThe surface energies of Cu(111) and Cu(100) at different CO* and OHˉ surface coverages.dA contour plot of the surface energy difference between Cu(100) and Cu(111) by changing the surface coverages of CO* and OHˉ.e, Wulff construction clusters of copper without and with (co-)adsorption of CO* and OHˉ. Accordingly, we found that the adsorption energy of OHˉ is more negative than that of CO* (Supplementary Table 1 ), indicating that OHˉ adsorption on Cu is more conducive to regulating the surface energy of the copper catalyst. Moreover, Cu(100) has a lower OHˉ adsorption energy than Cu(111) due to a lower coordination number of surface atoms. Additional electrons of OHˉ do not affect the dipole moment and magnetic property of Cu (Supplementary Fig. 7 and Supplementary Tables 2 – 4 ). The OHˉ adsorption therefore may not only decrease the surface energy of the system but also preferably promote the growth of Cu(100). The projected density of states about Cu(111) and Cu(100) with different *CO and OHˉ coverage were calculated to provide the electronic analysis for the adsorbates’ effect on surface energies. We found that the d band center of copper downshifts with increased adsorbate coverage (Supplementary Fig. 8 ), indicating that the *CO and OHˉ species could stabilize the surface. We then generated a surface energy difference (ΔE) map for Cu(111) and Cu(100) relating to CO* and OHˉ coverages (Fig. 1d ). We showed that with the buildup of CO&OHˉ co-adsorption, the growth of Cu(100) was prioritized relative to Cu(111) formation. We also carried out the Wulff construction calculation to estimate the ratio of Cu(100) and Cu(111) of a copper crystal with different coverages of CO* and OHˉ (Fig. 1e ). At CO* and OHˉ coverages of 4/9 ML, we obtained a 95% increase in the Cu(100) portion relative to copper without intermediates (Supplementary Table 5 ). Synthesis and characterizations of precatalyst and derived Cu catalyst Motivated by our DFT analysis, we sought to synthesize Cu(100)-rich catalysts with the aid of CO&OHˉ co-adsorption. To realize this, we turned our attention to phosphate anions, which bind strongly with Cu cations to form stable Cu complexes and can act as proton transport mediators to facilitate electrolysis [28] , [29] , [30] . We hypothesized that the electrochemical reduction of Cu precatalyst would be slowed by the addition of phosphate, which can promote the local proton concentration [29] and facilitate CO 2 R towards the co-production of CO* and OHˉ species; these active species adsorb easily at the positively charged Cu sites and thereby steer the Cu reconstruction to forming active Cu(100) facets (Fig. 1b ) [24] , [25] , [26] . Seeking experimentally to coordinate phosphate anions to Cu, we prepared a phosphate-doped copper oxychloride precatalyst using a sol-gel synthesis method. We modulated the P/Cu atomic ratio up to 0.6 in the Cu precatalysts by adjusting the concentrations of phosphate and copper precursors (Supplementary Fig. 9 and Supplementary Table 6 ), evidenced by energy-dispersive X-ray spectroscopy (EDX) and inductively coupled plasma optical emission spectroscopy (ICP-OES). Scanning transmission spectroscopy (SEM) and transmission electron microscopy (TEM) results showed that the precatalysts with or without phosphate showed a similar particle size of ~1 μm (Supplementary Figs. 10 – 12 ). To characterize the electronic structure of phosphate-containing Cu precatalyst, we carried out the Cu K-edge X-ray absorption spectroscopy (XAS) measurements. The X-ray absorption near edge structure (XANES) and its first derivative, Fourier-transformed extended X-ray absorption fine structure (EXAFS), together with the wavelet transform contour plot spectra suggested that the precatalyst exhibits a Cu structure akin to CuO (Fig. 2 a and b , Supplementary Fig. 13 ). The phosphate doping in the precatalyst was further evidenced by X-ray photoelectron spectroscopy (XPS, Supplementary Fig. 14 ). In addition, X-ray diffraction (XRD) and Fourier transform infrared spectroscopy (FTIR) results suggested that the phosphate-doped Cu precatalyst has a crystal structure matching the orthorhombic Cu 2 (OH) 3 Cl [31] , with the addition of phosphate ligands forming mono- or bidentate- complexes with the Cu cations (Fig. 2c , Supplementary Figs. 15 – 17 ). Fig. 2: Structural characterization of Cu precatalyst and derived Cu catalyst. The Cu K-edge XANES ( a ) and Fourier-transformed EXAFS ( b ) spectra of Cu precatalyst and standards (Cu foil, Cu 2 O, CuO, and Cu(OH) 2 ). c XRD spectra of precatalysts with and without phosphate and the relevant derived Cu catalysts after reduction; * and # represent diffraction peaks of Cu 2 (OH) 3 Cl and carbon paper substrate, respectively. Dark-field microscope images (left) and related SEM images (right) of Cu precatalyst after electrolysis at different reduction times, i.e. 0 min ( d ), 15 min ( e ), and 30 min ( f ). g Bright-field (top) and dark-field (bottom) TEM images of the Cu(100)-rich catalyst. Full size image Seeking to investigate the catalyst-evolution process, we spray-coated the precatalyst on a gas diffusion layer which was then fully reduced under CO 2 R conditions. The full reduction is evidenced by additional XPS analysis (Supplementary Fig. 18 ) and the color change of the electrode from green to metallic Cu red as seen in Raman microscope images (Fig. 2d–f ). Concurrently, the precatalyst underwent a dissolution-redeposition process, resulting in a significant morphological reconstruction from particles to cavities and dendrites. XRD and dark-field TEM results showed the predominant Cu(100) over Cu(111) facets in the resulting Cu catalyst (Fig. 2 c and g , Supplementary Fig. 19 ). By contrast, a Cu(111)-rich catalyst was obtained by reducing the phosphate-free Cu precatalyst under the same conditions (Fig. 2c , Supplementary Figs. 20 and 21 ). Additional electrochemical OHˉ adsorption measurements further indicate that Cu(100)-rich and Cu(111)-rich catalysts were derived from precatalysts with and without phosphate ligands, respectively (Supplementary Fig. 22a ). These results suggest that the addition of phosphate in the Cu precatalyst favors the growth of Cu(100) during CO 2 R and the portion of Cu(100) of derived Cu catalyst is increased by ~95% compared to that of a previous Cu catalyst synthesized in situ [13] (Supplementary Table 7 ) and that of the bare Cu control catalyst (Supplementary Figs. 15b and 22b, c , and Supplementary Table 8 ), consistent with our DFT simulations. In situ spectroscopic studies of catalyst evolution To gain molecular-level insights into the impact of phosphate ligands on Cu(100) formation, we conducted time-dependent in situ Raman experiments over the course of 30-min reduction time (Fig. 3a , Supplementary Figs. 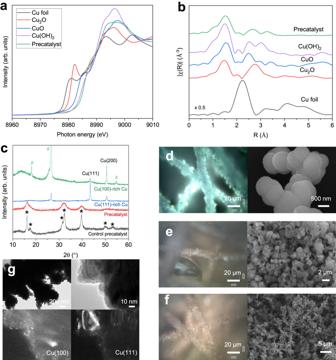Fig. 2: Structural characterization of Cu precatalyst and derived Cu catalyst. The Cu K-edge XANES (a) and Fourier-transformed EXAFS (b) spectra of Cu precatalyst and standards (Cu foil, Cu2O, CuO, and Cu(OH)2).cXRD spectra of precatalysts with and without phosphate and the relevant derived Cu catalysts after reduction; * and # represent diffraction peaks of Cu2(OH)3Cl and carbon paper substrate, respectively. Dark-field microscope images (left) and related SEM images (right) of Cu precatalyst after electrolysis at different reduction times, i.e. 0 min (d), 15 min (e), and 30 min (f).gBright-field (top) and dark-field (bottom) TEM images of the Cu(100)-rich catalyst. 23 and 24 ). For the phosphate-doped precatalyst, the intense peak at 298 cm −1 is attributed to the vibrations of the PO 4 3− group [32] . The phosphate peak intensity gradually decreased over the first 20 min. Concurrently, two new peaks at ~510 cm −1 and ~2060 cm −1 emerged at 3 min attributable to Cu-OH ad and CO* stretching, respectively [33] , [34] , and these two intense peaks persisted thereafter throughout the catalyst-evolving process. The high coverage of CO* at the catalyst surface was further verified by in situ attenuated total reflectance-surface enhanced infrared absorption spectroscopy (ATR-SEIRAS, Supplementary Fig. 25 ). By contrast, the phosphate-free precatalyst underwent a complete reduction within 10 mins with only weak OHˉ and CO* adsorptions present on Cu over this period (Fig. 3a ). This result supports the notion that phosphate doping slows the initial reconstruction of Cu and enables the enhanced co-adsorption of CO&OHˉ assisted by phosphate doping. Fig. 3: In situ spectroscopic interrogation. a – c In situ Raman spectra of Cu precatalyst evolution with (solid) and without (dot) phosphate collected in CO 2 -flowed 0.1 M KHCO 3 electrolyte at −1.1 V vs RHE; the shade areas represent the vibrations of the PO 4 3- group [32] . Time-dependent Cu K-edge XANES ( b ) and Fourier-transformed EXAFS ( c ) of Cu precatalyst with phosphate addition, the test was performed in CO 2 -flowed 0.1 M KHCO 3 electrolyte at −1.1 V vs. RHE over the course of 30-min reduction time; ocp stands for open-circuit potential. d The corresponding XANES fitting spectra in b , solid lines represent the experiment data and circles represent the linear combination fit spectra. e The percentage of metallic Cu at different reduction times. Values are extracted from linear combination fit using the XANES spectra of Cu precatalyst at ocp and metallic Cu as standards with the weighting factors as fit parameters. Coordination numbers (CN) of Cu-Cu (f) and Cu-O ( g ) at different reduction times extracted from the Cu K-edge EXAFS fittings (see Supplementary Table 10 ). Full size image To examine the catalyst formation process at an atomic level, we performed the time-dependent in situ Cu K-edge XAS experiments to monitor the dynamic changes of the Cu oxidation state and local coordination environment. During CO 2 R, the Cu precatalyst was fully reduced in 30 mins, in which the whiteline intensity gradually decreased whereas the pre-edge feature at ~8981 eV was progressively enhanced (Fig. 3b ). Two isosbestic points at 8995 eV and 9005 eV in the XANES region were observed, indicating a two-phase transformation from the Cu precatalyst to form a metallic Cu structure [35] , [36] . This finding is supported by EXAFS results (Fig. 3c ), in which the intensity of Cu–O bond slowly decreased with the emergence of metallic Cu-Cu bond. We then fit the XANES spectra using a linear combination method [14] , [19] , [37] (Fig. 3 d and e , Supplementary Table 9 ). We found that the catalyst evolution went through an exponential-like process: the Cu species underwent a rapid reduction at the first 15 mins corresponding to precatalyst dissolution (Fig. 2e , Supplementary Fig. 26 ); then at the catalyst redeposition stage, the Cu reduction assisted by co-adsorption of CO&OHˉ was relatively slow (Figs. 2 f and 3a , Supplementary Fig. 26 ). This was further confirmed by the EXAFS fitting results [37] , in which the formation of metallic Cu-Cu bond also followed an exponential-like trend (Fig. 3f , Supplementary Table 10 ). The covalent Cu-O coordination exhibited a steep reduction (Fig. 3g ), suggesting a relatively steady O-leaching from the precatalyst matrix during chronoamperometry electrolysis. We also performed in situ Cu K-edge XAS analysis of the control Cu precatalyst without phosphate (Supplementary Fig. 27 ); it shows a rapid Cu reduction compared to the Cu precatalyst with phosphate. These results also indicate that slow Cu reduction during catalyst redeposition process arises from strong noncovalent OHˉ adsorption on Cu [25] – an effect triggered by phosphate doping. These findings, taken together, illustrate that the addition of phosphate enables noncovalent interactions of Cu with OHˉ and CO* to prioritize the growth of Cu(100)-rich catalyst, promising more efficient C 2+ production. Electrochemical performance of CO 2 and CO reductions We evaluated the CO 2 R performance in a catholyte-free MEA electrolyzer with 0.1 M KHCO 3 flowing at the anode. Cu(100)-rich catalyst shows a peak FE C2+ of 83% at 500 mA cm −2 with a full-cell voltage of −3.8 V, translating to an EE C2+ of 25% and a C 2+ current density of 415 mA cm −2 (Fig. 4a ). This performance (EE × current) is double that of reported results in neutral MEA-CO 2 R systems (Supplementary Fig. 28 and Supplementary Tables 7 and 11 ), indicating the role of Cu(100)-rich sites in accelerating C-C coupling. The effect of electrochemical surface area (ECSA) on CO 2 R reactivity is not significant: Cu(100)-rich catalyst showed an ECSA value akin to Cu(111)-rich catalyst derived from a precatalyst without phosphate (Supplementary Fig. 29 and Supplementary Table 12 ). However, the Cu(100)-rich catalyst exhibited a 1.7× higher normalized C 2+ current density than the Cu(111)-rich catalyst, suggesting the intrinsic nature of activity improvement on Cu due to increased Cu(100). The Cu(100)-rich catalyst is stable, achieving a FE C2+ of 75% and an EE C2+ of 24% for initial 60 hours at 300 mA cm -2 (Fig. 4b ). Fig. 4: Electrochemical CO 2 /CO reduction performance of the Cu(100)-rich catalyst in a MEA electrolyzer. a FEs for all products at various current densities and related cell potentials from CO 2 reduction. b Extended CO 2 electrolysis using the Cu(100)-rich catalyst at 300 mA cm −2 . Operating conditions: 0.1 M KHCO 3 anolyte (pH ~8.4) at a flow rate of 20 mL min −1 and an average CO 2 inlet flow rate of ~75 sccm cm −2 at atmospheric temperature and pressure conditions, in which the catalyst loading is ~1 mg cm −2 . c FEs for all products at various current densities and related cell potentials from CO reduction. d FEs as well as SPCEs toward C 2+ products on the Cu(100)-rich catalyst at 500 mA cm −2 with different CO flow rates. e Extended CO electrolysis using the Cu(100)-rich Cu catalyst at 500 mA cm −2 . The Cu(100)-rich catalyst delivers an average FE C2+ of 86%, C 2+ current densities of 432 mA cm −2 , EE C2+ of 37%, and SPCE C2+ of 94% throughout. Operating conditions: 1 M KOH anolyte (pH ~14) at a flow rate of 20 mL min −1 and an average CO inlet flow rate of ~2 sccm cm −2 at atmospheric temperature and pressure conditions, in which the catalyst loading is ~1 mg cm −2 . Full size image Increasing CO and OHˉ concentrations in the catalyst layer would enhance the adsorptions of OHˉ and *CO [38] to facilitate C 2+ production on the Cu(100)-rich catalyst. Accordingly, we evaluated the performance of the Cu(100)-rich catalyst in the same MEA system by feeding CO gas at the cathode and flowing 1 M KOH at the anode: it shows a peak FE C2+ of 93% and a C 2+ current density of 465 mA cm −2 at −2.3 V, leading to an EE C2+ of 41% (Fig. 4c ). In situ Raman analysis (Supplementary Fig. 30 ) evidenced the co-adsorption of *CO&OHˉ at the catalyst with vastly increased OH − adsorption in the CO reduction system compared to the OH − adsorption during CO 2 electrolysis. This finding is consistent with our DFT results that additional OHˉ adsorption helps stabilize Cu(100) to accelerate C-C coupling. To advance SPCE C2+ in CO electrolysis, we decreased the areal flow rate of CO to 2 sccm cm −2 . At a current density of 500 mA cm −2 , we achieved an SPCE of 95% for C 2+ products (Fig. 4d ). The Cu(100)-rich catalyst is robust, delivering an average SPCE C2+ of 95%, a FE C2+ of 86%, an EE C2+ of 37%, and a C 2+ current density of 432 mA cm −2 for 150 hours (Fig. 4e ). This outperforms previously reported MEA-CO electrolysis systems with respect to EE × current (Supplementary Fig. 31 and Supplementary Table 13 ). In summary, this work presents a strategy to stabilize intermediates that facilitate Cu(100) growth during in situ catalyst materials synthesis. Using this strategy, we achieved efficient C 2+ productions from CO 2 /CO electrolysis with a high energy efficiency of 40% and a near-unity carbon efficiency. This performance is in the vicinity of industrial standards [20] , [39] and brings forward this technology in the direction of economic viability. Precatalyst preparation The precatalysts were fabricated by the following sol-gel method: first, copper (II) chloride dihydrate (CuCl 2 · 2H 2 O, 0.4104 g) was dissolved in 2 mL methanol, sodium hypophosphite (NaH 2 PO 2 ) in 2 mL methanol was also prepared in a separate vial, two solutions mentioned above were cooled in the freezer for 2 h. Next, NaH 2 PO 2 was then added dropwise to CuCl 2 · 2H 2 O. Then, 1 mL epoxypropane and a mixture of methanol and water (2 mL MeOH and 0.23 mL H 2 O) were slowly added under constant stirring resulting in a blue solution. The solution was then allowed to age at room temperature for more than three days to promote network formation and gelation. After aging, the gels were repeatedly washed and centrifuged with acetone three times and then dried under a vacuum for 24 hours. The precursors with different phosphorus-doped concentrations (NaH 2 PO 2 , 0.0306, 0.0918, and 0.1530 g) were synthesized by changing the amount of NaH 2 PO 2 and were denoted as CuP0.2, CuP0.4, and CuP0.6, respectively. As a control, the precursor without phosphorus was also synthesized, labeled CuP0. Electrode preparation To prepare the deposition ink, 20 mg of the precursor was dispersed in a mixture of 0.95 mL 2-propanol, and 50 μL 5 wt% Nafion solution (Sigma-Aldrich) and then sonicated for at least 1 hour. The ink was air-brushed onto 2 × 4 cm carbon paper (Toray TGP-H-060 with an MPL layer) with the loading of ~1 mg/cm 2 and dried to form the copper sol-gel working electrode. The loading was determined by measuring the weight of the carbon paper before and after deposition. CO 2 R in flow-cell The CO 2 R activity of the catalysts was investigated by performing electrolysis in a two-compartment flow-cell configuration using a 1.0 M KOH electrolyte. The three-electrode set-up was connected to a potentiostat (Autolab 204). Flow-cell configuration consists of catalysts spray-coated gas diffusion layer as the cathode, an anion exchanged membrane (AEM, Fumasep FAA-3-PK-130) as the membrane, and NiFe/Ni foam as the anode, Ag/AgCl was used as the reference electrode. CO 2 gas flowed behind the gas diffusion layer at a rate of 50 mL/min. The performance of the cathode was evaluated by performing constant-current electrolysis. Gas products were routed into a gas chromatograph with a thermal conductivity detector and a flame ionization detector (GC-2060A). Nitrogen (99.999%) was used as the carrier gas. 1 H NMR spectrum (Bruker, AVANCE IIITM HD 400 MHz) was used to determine the liquid products in 10% D 2 O using water suppression mode, for which dimethyl sulfoxide was added as an internal standard. All the electrode potentials were converted to values regarding the RHE using the following equation: 
    E_RHE=E_Ag/AgCl+0.197V× 0.0591×pH+85%  i R
 (1) The ohmic loss between the working and reference electrodes was measured using the electrochemical impedance spectroscopy technique (with frequency ranges from 100 kHz to 0.1 Hz and amplitude of 10 mV.) and 85% iR compensation ( i is the current density, R is the uncompensated resistance) was applied to correct the potentials manually. CO 2 R/COR in MEA electrolysers The CO 2 R and COR experiments were performed in a membrane electrode assembly (MEA) using neutral (0.1 M KHCO 3 ) and alkaline (1 M KOH) media electrolytes, respectively. The performance tests were conducted using an electrochemical test station. The test station was equipped with the components, including a commercial MEA electrolyzer, a current booster (Metrohm Autolab, 10A), a mass flow controller (Sierra, SmartTrak 100), a humidifier, an electrolyte container, and a peristaltic pump with silicon tubing. 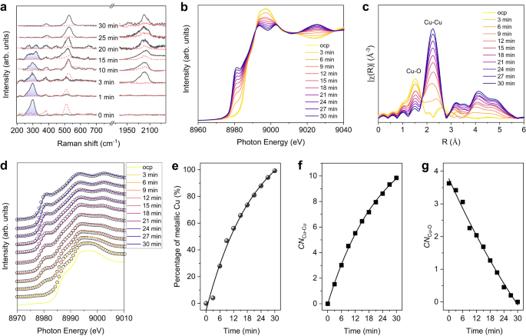Fig. 3: In situ spectroscopic interrogation. a–cIn situ Raman spectra of Cu precatalyst evolution with (solid) and without (dot) phosphate collected in CO2-flowed 0.1 M KHCO3electrolyte at −1.1 VvsRHE; the shade areas represent the vibrations of the PO43-group32. Time-dependent Cu K-edge XANES (b) and Fourier-transformed EXAFS (c) of Cu precatalyst with phosphate addition, the test was performed in CO2-flowed 0.1 M KHCO3electrolyte at −1.1 V vs. RHE over the course of 30-min reduction time; ocp stands for open-circuit potential.dThe corresponding XANES fitting spectra inb, solid lines represent the experiment data and circles represent the linear combination fit spectra.eThe percentage of metallic Cu at different reduction times. Values are extracted from linear combination fit using the XANES spectra of Cu precatalyst at ocp and metallic Cu as standards with the weighting factors as fit parameters. Coordination numbers (CN) of Cu-Cu (f) and Cu-O (g) at different reduction times extracted from the Cu K-edge EXAFS fittings (see Supplementary Table10). 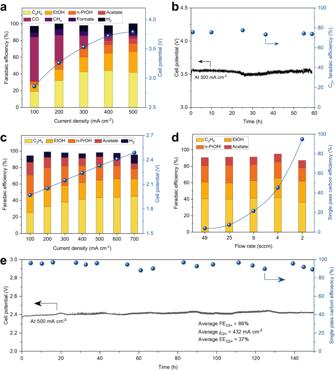Fig. 4: Electrochemical CO2/CO reduction performance of the Cu(100)-rich catalyst in a MEA electrolyzer. aFEs for all products at various current densities and related cell potentials from CO2reduction.bExtended CO2electrolysis using the Cu(100)-rich catalyst at 300 mA cm−2. Operating conditions: 0.1 M KHCO3anolyte (pH ~8.4) at a flow rate of 20 mL min−1and an average CO2inlet flow rate of ~75 sccm cm−2at atmospheric temperature and pressure conditions, in which the catalyst loading is ~1 mg cm−2.cFEs for all products at various current densities and related cell potentials from CO reduction.dFEs as well as SPCEs toward C2+products on the Cu(100)-rich catalyst at 500 mA cm−2with different CO flow rates.eExtended CO electrolysis using the Cu(100)-rich Cu catalyst at 500 mA cm−2. The Cu(100)-rich catalyst delivers an average FEC2+of 86%, C2+current densities of 432 mA cm−2, EEC2+of 37%, and SPCEC2+of 94% throughout. Operating conditions: 1 M KOH anolyte (pH ~14) at a flow rate of 20 mL min−1and an average CO inlet flow rate of ~2 sccm cm−2at atmospheric temperature and pressure conditions, in which the catalyst loading is ~1 mg cm−2. The MEA setup consisted of titanium anode and stainless-steel cathode flow-field plates with geometric flow-field areas of 1 cm 2 . The MEA was composed of three components: a cathode electrode (as described earlier), an anode electrode (IrO x supported on a titanium (Ti) felt (Fuel Cell Store)), and an anion exchange membrane (AEM, Sustainion® X37-50). The cathode and anode electrodes were separated from each other using an AEM. The AEM was rinsed with DI water for 15 min before performance testing. The MEA was assembled by a compression torque applied to the each of associated bolts. The cathode flow field was used for the supply of humidified CO 2 /CO over the backside of the cathode gas diffusion electrode, whereas the anode flow field was used for the supply of anolyte through the anode electrode. The IrOx-Ti electrode was prepared by following a procedure involving several steps: (1) immersing the Ti felts into a homogenous ink of 2-propanol, iridium (IV) chloride dehydrate (Premion®, 99.99%, metal basis, Ir 73%, Alfa Aesar), and hydrochloric acid (HCl), (2) drying the resulting electrodes at 100 °C for 10 min and sintering the dried electrodes at 500 °C for 10 min, and (3) repeating the first two steps until an IrO x mass loading of 1 mg/cm 2 . After the MEA assembly, the anolyte (0.1 M KHCO 3 for CO 2 R and 1 M KOH for COR) was fed into the anode flow field, and the humidified gaseous reactant (CO 2 for CO 2 R and CO for COR) was fed into the cathode flow field. A constant current density of 100 mA cm −2 was applied to initiate the CO 2 R or COR, and the current density was gradually increased with 100 mA cm −2 increments. The current increments were made after stabilization of the cell potential, which typically required 30-40 minutes. At each current density, gas products of CO 2 R or COR were analyzed using gas chromatography (GC). The liquid products of CO 2 R or COR were collected from the cathodic and anodic downstream simultaneously. CO 2 R/COR product analysis The Faradaic efficiency of gas products was calculated as follows. Faradaic  efficiency(%)=N× F×ν× r/(i×V_m)
 (2) where N represents the number of electrons transferred, F represents the Faradaic constant, v represents the gas flow rate at the cathodic outlet, r represents the concentration of product(s) in ppm, i represents the total current, and V m represents the unit molar volume of product(s). The gas flow rate at the cathode outlet was measured via a bubble flow meter. The liquid products of CO 2 R or COR were analyzed by using 1 H NMR spectroscopy (600 MHz Agilent DD2 NMR Spectrometer) with suppressing water peak. Dimethyl sulfoxide (DMSO) was used as the reference standard, whereas deuterium oxide (D 2 O) was used as the lock solvent. The NMR spectra collected at each current density were used to calculate the Faradaic efficiency toward liquid products of CO 2 R or COR as follows. Faradaic  efficiency(%)=N× F×n_product/Q
 (3) where N represents the number of electrons transferred, F represents the Faradaic constant, n product represents the total mole of product(s), and Q = i × t represents the total charge passing during the liquid product collection. Energy efficiency (EE) calculation The full-cell energy efficiencies toward CO 2 R or COR products were determined as follows. EE_product=E_cell^o/E_cell×FE_product× 100%
 (4) 
    E_cell^o=ΔG^o/-zF
 (5) where \({E}_{{cell}}^{o}\) represents the thermodynamic cell potential for CO 2 R or COR products, \(\Delta {G}^{o}\) represents the change in Gibbs free energy, and E cell represents the applied cell voltage ( iR -free). Single-pass carbon efficiency (SPCE) calculation SPCE toward gas, liquid, or a group of gas and liquid products of COR (at 25 ◦ C and 1 atm) was calculated as follows. SPCE=(j× 60)/(N× F)/(flow  rate(L/min )× 1(min ))/(24.05(L/mol))
 (6) where j represents the partial current density toward a COR product, N represents the number of electrons transferred to produce 1 mole of product. Material characterization The phase of catalyst powder was verified by XRD with a Bruker D8 Advanced diffractometer using Cu Kα radiation (λ = 1.5406 Å). The surface morphology and composition of the catalysts were characterized by scanning electron microscopy (SEM, JEOL JSM-7800F) instruments with energy-dispersive X-ray spectroscopy (EDX). Transmission electron microscope (TEM), high-resolution TEM (HRTEM), and TEM-mapping images were performed on a JEOL JEM-2100F operated at 200 kV. To obtain the dark-field TEM images for the Cu(100)-rich catalyst, we first carried out selected area electron diffraction, then trapped the diffraction spots on the specific crystal facets using the aperture slot, and finally took the dark field photographs. X-ray photoelectron spectroscopy (XPS) for surface element investigation before and after CO 2 R was carried out by using a Thermo Scientific K-Alpha+ source XPS system. Inductively coupled plasma optical emission spectroscopy (ICP-OES, Thermo iCAP7000) was carried out to determine the contents doped into copper in precursor, 5 mg of the sample was completely dissolved into 1 L deionized water with 5 mM HNO 3 and sonicated for 30 min for the ICP-OES test. In situ X-ray absorption spectroscopy (XAS) measurements We performed the in situ Cu K-edge XAS measurements at the Beamline BL11B of the Shanghai Synchrotron Radiation Facility and the SuperXAS beamline of the Swiss Light Source, Villigen, Switzerland. The in situ XAS setup is akin to our previous report [19] . Fluorescence X-ray signals were recorded. During measurements, XAS spectra were recorded at a time resolution of 1 s, which were then averaged for X-ray absorption near-edge spectra (XANES) and extended X-ray absorption fine structure (EXAFS) analyses. Aqueous 0.1 M KHCO 3 electrolytes were flowing at both the anode and cathode compartments, which were separated by an anion-exchange membrane (AEM, Fumasep FAA-3-PK-130). An Ag/AgCl (saturated KCl) and a sputtered Pt on carbon paper were used as reference and counter electrodes, respectively. A Cu precatalyst loaded on carbon paper was the working electrode. An electrochemical workstation (Gamry Interface 1000) was used to power the test. XAS analysis XAS data were processed with Demeter (v.0.9.26). We performed The XAS spectral normalization was performed using Athena software in Demeter, in which a cubic spline function was used to fit the background above the absorption edge [40] . We then applied Fourier transformation of the EXAFS spectra from an energy (E) space to a radial distance (R) space. We fit EXAFS spectra using Artemis software in Demeter with the FEFF6 program. Data range k = 3-11 Å −1 , amplitude reduction factor \({S}_{0}^{2}\) = 0.8. The coordination numbers (N) were fixed to the expected values listed in cif files of Cu 2 (OH) 3 Cl and Cu foil, bond distances (R) and the Debye Waller factor (σ 2 ) for each cell were determined. Then the Debye Waller values were fixed to calculate N. In situ Raman tests In-situ Raman experiments were performed using a Renishaw inVia Raman microscope in a homemade CO 2 -saturated 0.1 M KHCO 3 aqueous solution as the electrolyte. The signals were collected using a water-immersion objective at the excitation laser source of 633 nm. In situ Attenuated total reflection-surface-enhanced infrared absorption spectroscopy (ATR-SEIRAS) tests ATR-SEIRAS were measured using a Thermo Scientific Nicolet iS50 FTIR Spectrometer with a Pike VeeMAX III attachment. 10 mg of the precursor was dispersed in a mixture of 0.95 mL 2-propanol, and 50 μL 5 wt% Nafion solution (Sigma-Aldrich) and sonicated for 30 min, then drop coated on Au film. Spectra were recorded at a resolution of 4 cm −1 in a CO 2 − saturated 0.1 M KHCO 3 -D 2 O electrolyte. Electrochemical OH - adsorption and ECSA evaluation Electrochemical OH - adsorption was performed in an N 2 -saturated 1.0 M KOH electrolyte with a linear sweep voltammetry method at a sweep rate of 100 mV/s for copper. The potential ranged from −0.2 to 0.6 V vs RHE. The electrochemical active surface area (ECSA) was measured by using double-layer capacitance and determined based on the equation ECSA = R f S, where R f was the roughness factor and S was the geometric area of the electrode (1 cm −2 ). R f = C dl /0.034, where C dl was the double-layer capacitance of catalysts and 0.029 mF/cm 2 was the double-layer capacitance of a smooth Cu foil [12] . All the catalysts were scanned at a non-Faradaic region of −0.06 to −0.02 V vs RHE, in N 2 -saturated 1.0 M KOH for ten cycles at sweep rates of 40, 60, 80, and 100 mV s −1 . DFT calculations DFT calculations were performed using the Vienna ab initio Software (VASP) [41] , [42] , Vander Waals interactions were accounted for by using the DFT-D3 method [43] . The generalized gradient approximation (GGA) with Perdew, Burke, and Ernzerh (PBE) functional is adopted to describe the electron exchange-correlation interaction [44] , [45] . Electron wave functions are expanded in plane waves with a kinetic energy cutoff of 400 eV. The method of Methfessel-Paxton (MP) with a smearing width of 0.20 eV was employed to transition metal surfaces and interfaces [46] . The convergence criterion for the electronic self-consistent iteration and force was set to 10 –5 eV and 0.05 eV Å −1 , respectively. A vacuum layer of 15 Å was introduced to avoid the interactions between periodic images. (3 × 3 × 1) k-point grid was used as these models. To evaluate the stability of one surface, the surface energy was used as defined below [47] : 
    E_surface=E_total-nE_ref-E_ads/2A
 (7) Where E total is the total energy of this surface from DFT calculations; E ref is the reference energy of unit composition from bulk calculations; E ads is the sum of the adsorption energies of the intermediates/molecular at given coverages; A is the surface area; and n is the number of unit composition in this surface, the less stable this surface is. For each coverage of the model, the most stable configuration was selected manually. In this work, the adsorbed molecule is CO* and OH - . To simulate the charge of OH − , additional valence electrons were added to the model, which is equal to the number of OH − . Surface energies with adsorption of two intermediates states were calculated by assuming that there were no adsorbate-adsorbate interactions [48] . The energy of CO* and OH - is obtained by the equation below: 
    E_molecular=E_scf+ΔZPE-TΔ S+∫_0^298.15KC_pdT
 (8) Where the E SCF is the electronic SCF energies from DFT, ΔZPE is the zero-point energy and TΔS is the entropy correct. The entropy and heat capacity corrections are evaluated. For the gas molecules, rotational and translational entropies were included in addition to vibrational entropies.